Nanoconfinement effects on hydrated excess protons in layered materials Thin water layers confined between surfaces are known for their surprising properties. Layered minerals, such as mackinawite, are naturally occurring systems where water is known to intercalate. Here we report, based on ab initio simulations, how excess protons can be hosted by the resulting nanostructured water film depending on the mackinawite interlayer distance. Even extreme nanoconfinement due to the mackinawite sheets is shown to not affect the dynamical nature of the topological defect, thus not localizing the excess protons but rather conserving the efficient structural (Grotthuss) diffusion process known in bulk water. Yet, depending on the width of the slit pore, the defect can bridge the bilayer water structure, thus forcing the excess proton into the water-depleted region between the bilayers. Confined liquids exhibit very different structural and dynamical properties compared with those of the corresponding bulk systems. Especially nanoconfined water, being of ubiquitous importance from biology to materials science, has been widely studied in both wire-like [1] , [2] , [3] , [4] and two-dimensional [5] , [6] , [7] , [8] environments. A feature of particular interest in such systems is the behaviour of excess protons. The solvated excess proton in bulk water has been widely studied using computer simulations and is now broadly understood [9] , [10] , [11] , [12] , [13] . In recent years, great progress has also been made in the understanding of excess protons in confined water. However, almost all efforts in this field are devoted to studying excess protons and proton transfer in water wires [14] , [15] , [16] , [17] , [18] , [19] , [20] owing to the importance of water channels in biological systems [21] , [22] , [23] , [24] and in view of technological applications such as fuel cells [25] , [26] , [27] , whereas investigations of hydrated protons at liquid/solid interfaces [28] , [29] , [30] are scarce. Here, we address the behaviour of excess protons in nanoconfined water between sheets of mackinawite minerals [31] , FeS, which form layer-like superstructures. Recently, precipitated mackinawite has been obtained under conditions of submarine alkaline hydrothermal vents [32] , thus making mackinawite minerals a very plausible medium for facilitating prebiotic synthesis as proposed in the ‘iron-sulphur world’ hypothesis [33] , [34] . Within this scenario, structures consisting of mackinawite layers with intercalated water at elevated temperature and pressure conditions, about 500 K and 20 MPa, are ideally suitable nanoreactors for such prebiotic processes. Indeed, it has been demonstrated that the structural and dynamical properties of the confined water lamella are dramatically dependent on the interlayer distance [35] , thus offering rich confinement effects on subsequent processes. Although sufficiently small intersheet distances lead to ‘arrested water’, such larger distances support liquid-like dynamics, where a stratified structure consisting of two water layers parallel to the FeS mineral surfaces is adopted with a low-density region separating them. Clearly, such nanostructured water films confined by real mineral surfaces will strongly impact any process occurring therein, proton hydration and transfer being the most paradigmatic and generic ones. Exploring this issue, which is the focus of the present study, is of immediate importance to such diverse fields as materials science, chemical physics and geophysics, to name but a few. Our main finding is that excess proton transfer in two-dimensionally confined water layers is an essentially barrierless process at the studied conditions, and that the excess proton is even capable of crossing water-depleted regions separating well-defined water layers parallel to the confining surfaces. Density profiles The core question to be addressed in the following relates to the structure and localization of an excess proton in thin water layers that are nanoconfined by FeS mineral surfaces. We study two lamellae setups: narrow (N) and wide (W), as depicted by representative snapshots in panels a/b and c/d of Fig. 1 , respectively. The resulting total density, resolved in terms of oxygen and hydrogen sites, is depicted in Fig. 2 (dotted lines), where the distinctly different density profile of the narrow slit pore system N ( Fig. 2a ) compared with system W ( Fig. 2b ) is readily visible. These total density profiles in both systems are virtually indistinguishable from those determined earlier for neutral water [35] , that is, the excess proton does not affect the overall structure of the water lamellae. 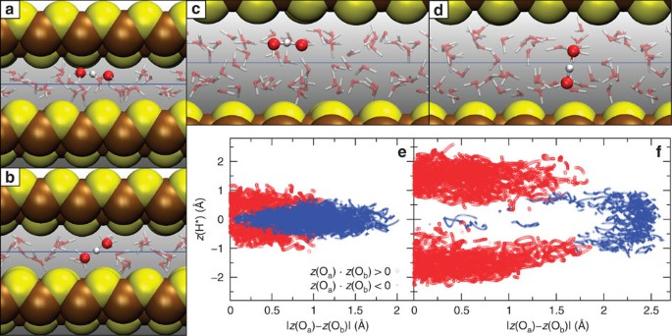Figure 1: Orientation and configuration map of the protonic defect. (a–d) Representative configuration snapshots of the protonic charge defect (highlighted by large spheres that mark the most active hydrogen bond, OaH*Ob, see text) in system N (a,b) and system W (c,d); the horizontal blue lines mark thez=0 Å midplane and the Fe, S, O and H atoms are indicated by brown, yellow, red and grey spheres, respectively. (e,f) Configuration map of the defect as a function ofz(H*) and |z(Oa)−z(Ob)| for system N (e) and system W (f); see text for the definitions ofz, H*, Oaand Ob. Within this plane, the red symbols distinguish those configurations where both oxygen sites of the charge defect are on one side of the midplane (cf. snapshotsaandc) from those where the defect reaches across the midplane in blue (cf. snapshotsbandd). The charge defect is oriented parallel to the mineral surface in the limit |z(Oa)−z(Ob)|=0, whereas higher values of |z(Oa)−z(Ob)| imply a pronounced inclination with respect to the surface. Figure 1: Orientation and configuration map of the protonic defect. ( a – d ) Representative configuration snapshots of the protonic charge defect (highlighted by large spheres that mark the most active hydrogen bond, O a H*O b , see text) in system N ( a , b ) and system W ( c , d ); the horizontal blue lines mark the z =0 Å midplane and the Fe, S, O and H atoms are indicated by brown, yellow, red and grey spheres, respectively. ( e , f ) Configuration map of the defect as a function of z (H*) and | z (O a )− z (O b )| for system N ( e ) and system W ( f ); see text for the definitions of z , H*, O a and O b . Within this plane, the red symbols distinguish those configurations where both oxygen sites of the charge defect are on one side of the midplane ( cf . snapshots a and c ) from those where the defect reaches across the midplane in blue ( cf . snapshots b and d ). The charge defect is oriented parallel to the mineral surface in the limit | z (O a )− z (O b )|=0, whereas higher values of | z (O a )− z (O b )| imply a pronounced inclination with respect to the surface. 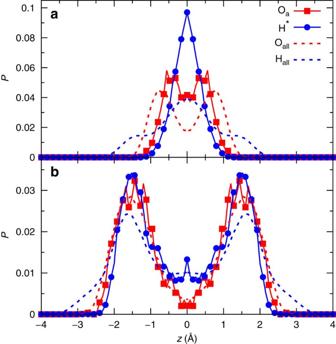Figure 2: Density profiles. Normalized density profilesP(z) along thecaxis, that is, normal to the confining surfaces, wherez=0 Å defines the midplane, for the specific protons and oxygens, H* and Oa(solid lines), of the excess charge defect (see text for definitions), as well as for all H and O sites for comparison (dotted lines) for system N (a) and system W (b). The distributions are symmetrized at the midplane to account for the underlying symmetry. Full size image Figure 2: Density profiles. Normalized density profiles P ( z ) along the c axis, that is, normal to the confining surfaces, where z =0 Å defines the midplane, for the specific protons and oxygens, H* and O a (solid lines), of the excess charge defect (see text for definitions), as well as for all H and O sites for comparison (dotted lines) for system N ( a ) and system W ( b ). The distributions are symmetrized at the midplane to account for the underlying symmetry. Full size image Free energy barriers Next, the free energy profile for proton transfer, Δ F ( δ ), is obtained by considering the proton transfer order parameter, that is, the asymmetric stretch coordinate of the so-called ‘most active hydrogen bond’ [36] (obtained from the O a H*O b triple, with the smallest | δ | value in a given configuration where O a is the oxygen of the H 3 O + protonic defect that has three closest protons attached to it; the corresponding donor−acceptor distance, O a ...O b , is denoted by R OO ). First, no significant differences in the profiles are observed between the N and W lamellae setups according to Fig. 3 . Second, comparing the free energy barrier for proton transfer in the lamellae with that in protonated bulk water at the same thermodynamic conditions reveals that even extreme confinement, such as realized in the narrow system N, does not hinder proton transfer compared with the bulk phase. Moreover, all free energy profiles are considerably flatter than in bulk water at 300 K, where a thermal barrier of about 1 k B T has been found [36] , [37] . Such a practically negligibly low free energy barrier for proton transfer as a result of purely thermal activation is consistent with similar results reported on confined water wires [18] , [20] . One is thus tempted to speculate that, in general, confinement effects on water, even extreme ones, such as those realized by squeezing water as much as in system N, do not lead to the localization of excess protons. On the contrary, such two-dimensional nanoconfinement by mineral surfaces rather supports the same efficient structural (Grotthuss) diffusion process of defect charges as it is known from the bulk phase. Indeed, it would be highly interesting to probe the possible impact of excess protonation on the anomalous behaviour suggested for protons in nanoconfined water, as it has been extracted from deep inelastic neutron scattering [2] , [38] . 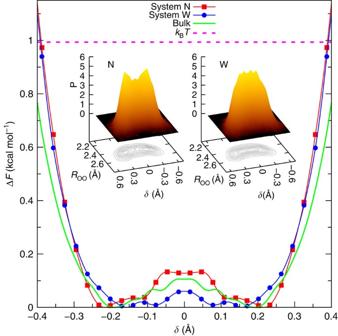Figure 3: Free energies. Free energy profiles, ΔF(δ), for the transfer of the excess proton along the most active hydrogen bond (see text) in system N (red squares), W (blue circles) and in the bulk (solid green line) at 500 K; the thermal energykBT≈1 kcal mol−1is marked by a horizontal dashed line. The corresponding two-dimensional distribution functions,P(δ,ROO), are shown in insets N and W, respectively. The data are smoothened for presentation. Figure 3: Free energies. Free energy profiles, Δ F ( δ ), for the transfer of the excess proton along the most active hydrogen bond (see text) in system N (red squares), W (blue circles) and in the bulk (solid green line) at 500 K; the thermal energy k B T ≈1 kcal mol −1 is marked by a horizontal dashed line. The corresponding two-dimensional distribution functions, P ( δ , R OO ), are shown in insets N and W, respectively. The data are smoothened for presentation. Full size image Structure of the protonic defect In water, it has been well established that protonic defects are the most ‘fluxional complexes’ [36] , rather than well-defined structural species [9] , [10] , [11] , [13] . In the insets of Fig. 3 , the shape of the distribution function P ( δ , R OO ) indicates that the protonic defect adopts a wide range of structures in both lamellae in the same way as it happens in bulk water. Moreover, the limiting structures [36] characterized by | δ |≤0.1 and | δ |>0.3 (that is, the so-called idealized ‘Zundel’ and ‘Eigen’ complexes, respectively) have the same structural features in these strongly confined systems as in bulk water [37] (which is revealed by comparing their radial distribution functions, data not shown). In conclusion, the confined excess protons compare extremely well with the dynamical nature of protonic defects in liquid water [36] in terms of rapid thermal interconversion between Eigen-like and Zundel-like structures, which underlies the adiabatic proton transfer concept, the structural (Grotthuss) diffusion mechanism and thus the anomalously large diffusion coefficient [9] , [10] , [11] , [13] . Again, the nanoconfinement established by narrow mineral surfaces does not lead to any confinement of the protonic defects. Location and orientation of the protonic defect The density profiles of the protonic charge defect as characterized by H* and O a , see the solid lines in Fig. 2 , largely follow those of the water molecules (see dotted lines therein), which are distinctly different in the N and W lamellae, namely pronounced unimodal and bimodal, respectively. This shows that the charge defects must nicely integrate in the sense of topological defects into the confined hydrogen bonding network akin to what is known from the bulk environment [9] , [10] , [11] , [13] . In the narrow slit pore, however, the water molecules point with their hydrogens towards the mineral surface, whereas the oxygen sites are closer to the confining surface than in case of the H 3 O + defect. A similar, albeit much weaker effect is also observed for the wider lamella. Do these seemingly subtle differences herald a preferred orientation of excess protons at the water/mineral interface? Indeed, despite the fact that confinement does not affect the structure of the hydrated Zundel/Eigen complex as such, the representative snapshots of the charge defects in Fig. 1 point towards distinct orientations that are preferred in the narrow and wide lamellae, respectively. In the case of the narrow pore, the distribution in Fig. 1e clearly reflects the density profile from Fig. 2 . Analysis of the configurations reveals that about 70% of the arrangements are such that the two ends of the defect’s hydrogen bond, that is, the oxygen ends of the O a H*O b triple, are on different sides of the midplane. Overall, there is not much orientational correlation within the narrow pore (as shown by the overlap of the red and blue points in Fig. 1e ) as the defect lies essentially flat within the compressed water layer. In stark contrast, a significant influence on defect arrangement within the nanopore is recognized in system W, which depends on both its position with respect to the midplane, as measured by z ( H *), and the orientation of the hydrogen bond axis w.r.t. the midplane, which is quantified by | z (O a )– z (O b )|. Analysis shows that, here, about 20% of all defect configurations bridge the water bilayer, thus pushing the excess proton into the water-depleted region at the centre of the pore as represented in Fig. 1d , whereas the defect lies flat and fully embedded within one of the two bilayers in 80% of the cases. Regarding possible correlations between the orientation of the protonic defect and its local structure, we analysed the ratio of Zundel versus Eigen structures depending on the orientation but found no meaningful correlations between them. The data shown in Figs 1 and 2 , as well as the lack of correlation between the Zundel/Eigen ratio and the orientation of the protonic defect, lead to the same conclusion for both systems N and W. The confinement imposes a particular nanostructure of the water layer and consequently also a particular arrangement of the hydrogen bond network in which the excess proton exists as a dynamical topological defect, much in the same way as it happens in bulk water. In consequence, although the confinement has a strong effect of imposing a particular arrangement of the topological defect with respect to the confining surfaces depending on the width of the pore, surprisingly, the local structure of the excess proton as such is not significantly affected by the confinement. In particular, the confinement stabilizes neither Zundel nor Eigen structures, even in the narrow pore limit N, but the excess proton still exists as a dynamical defect much like in the bulk. Thus, these ab initio simulations of nanoconfined acidic water between sheets of a mackinawite FeS mineral reveal very efficient proton transfer. As in bulk water, the excess proton can be considered as a dynamical charge defect even at extreme confinement, being fully incorporated into the hydrogen bond network as a topological defect. The transfer of this excess proton along the hydrogen bond network is an almost barrierless process, which implies most efficient proton migration even at nanoconfinement conditions. Our findings not only suggest that, indeed, thin water films confined by such mineral sheets are efficient nanoreactors for prebiotic reactions in nature, but they might also lead to the design of improved setups for fuel cell membranes. Computational approach The methods and system set-up are the same as those that have been carefully tested and validated in our previous investigation of pure water confined between mackinawite sheets [35] . Thus, the Perdew−Burke−Ernzerhof density functional [39] , [40] , together with ultrasoft pseudopotentials [41] (containing d -projectors in the case of sulphur and semicore states as well as scalar relativistic corrections for iron), at a plane wave cutoff of 25 Ry is used. The ab initio molecular dynamics simulations [42] are performed with the Car−Parrinello algorithm as implemented in the CPMD package ( http://www.cpmd.org ) [43] . Massive Nosé−Hoover chains thermostats [44] were applied to both nuclei and electrons together with a fictitious orbital mass of 700 a.u., a timestep of 2 a.u., substituting D for H masses, and using a high-order Suzuki−Yoshida algorithm to properly integrate the equations of motion of the thermostats; test runs of system N using orbital masses of 500 and 900 a.u. yielded similarly stable Car−Parrinello propagation. The systems were equilibrated for 5 ps before starting the production runs for another 24 ps. Model systems The crystal structure of mackinawite [31] consists of a tetragonal unit cell of Fe 2 S 2 with lattice parameters a = b =3.6795 Å and c =5.030 Å. The structure is layered and can be easily cleaved, thereby exposing the (001) surfaces. We employ a supercell consisting of 64 Fe and S atoms arranged in two Fe 32 S 32 parallel layers with which we design two systems. In system N (narrow), the layers are situated at the top and bottom of a supercell with c =13.82 Å, so that the neighbouring layers of adjacent supercells keep the ideal spacing of 5.03 Å. System W (wide) is analogous to N but with c =16.73 Å, and in both systems the ideal a = b values are kept. The topmost and bottommost S atoms are frozen at their ideal positions. The empty interlayer spaces at the centre of these two supercells are filled with 32 and 49 H 2 O molecules for system N and W, respectively. Adding an excess proton to each one of them yields the narrow and wide lamellae set-ups as depicted by representative snapshots in panels a/b and c/d of Fig. 1 , respectively. At the simulation temperature of 500 K, this yields a pressure of roughly 20 MPa according to the experimental data, chosen as to mimick typical hydrothermal vent conditions [35] . As a consistent reference, a protonated bulk water system containing 32 H 2 O molecules and an excess proton in a cubic supercell with a =10.415 Å was simulated with the same computational approach and parameter settings. Electronic structure analyses The electronic properties of the protonated water/mineral interfaces have been carefully analysed in terms of bonding charge, projected density of states and Löwdin charge analyses using representative configurations sampled from independent parts of the trajectories of both the wide and narrow lamellae. All these data show that there is essentially no charge transfer from FeS into the protonated water layers; note that the mineral slabs are internally polarized owing to the presence of protonated water, which results in negative charge accumulation inside the mineral and close to the interface with water. The interactions at this liquid−solid interface are limited to (time- and space-) local induced polarization of the mineral surface due to the water and/or hydronium dipoles in the fluctuating hydrogen bond network much in the same way as found earlier for neutral water [35] ; in particular, there is no excess correlation between the position of the cationic defect at the contact plane and accumulation or depletion of negative charge at the surface. How to cite this article: Muñoz-Santiburcio, D. et al. Nanoconfinement effects on hydrated excess protons in layered materials. Nat. Commun. 4:2349 doi: 10.1038/ncomms3349 (2013).